Regional climate impacts of a possible future grand solar minimum Any reduction in global mean near-surface temperature due to a future decline in solar activity is likely to be a small fraction of projected anthropogenic warming. However, variability in ultraviolet solar irradiance is linked to modulation of the Arctic and North Atlantic Oscillations, suggesting the potential for larger regional surface climate effects. Here, we explore possible impacts through two experiments designed to bracket uncertainty in ultraviolet irradiance in a scenario in which future solar activity decreases to Maunder Minimum-like conditions by 2050. Both experiments show regional structure in the wintertime response, resembling the North Atlantic Oscillation, with enhanced relative cooling over northern Eurasia and the eastern United States. For a high-end decline in solar ultraviolet irradiance, the impact on winter northern European surface temperatures over the late twenty-first century could be a significant fraction of the difference in climate change between plausible AR5 scenarios of greenhouse gas concentrations. The past few decades have been characterized by a period of relatively high solar activity. However, the recent prolonged solar minimum and subsequent weak solar cycle 24 have led to suggestions that the grand solar maximum may be at an end [1] . Using past variations of solar activity measured by cosmogenic isotope abundance changes, analogue forecasts for possible future solar output have been calculated. An 8% chance of a return to Maunder Minimum-like conditions within the next 40 years was estimated in 2010 (ref. 2 ). The decline in solar activity has continued, to the time of writing, and is faster than any other such decline in the 9,300 years covered by the cosmogenic isotope data [1] . If this recent rate of decline is added to the analysis, the 8% probability estimate is now raised to between 15 and 20%. A number of studies have indicated that the decreases in global mean temperature associated with a future decline in solar activity are likely to be relatively small [3] , [4] , [5] , [6] , [7] . However, variability in ultraviolet solar irradiance has been linked to changes in surface pressure that resemble the Arctic and North Atlantic Oscillations (AO/NAO) [8] , [9] , [10] and studies of both the 11-year solar cycle [11] , [12] and centennial timescales [13] suggest the potential for larger regional effects. The mechanism for these changes is via a stratospheric pathway, a so-called ‘top-down’ mechanism, and involves altered heating of the stratosphere by solar ultraviolet irradiance. Anomalous temperatures in the region of the tropical stratopause give rise to changes in the subtropical stratospheric winds, in geostrophic balance with the modified equator-to-pole temperature gradient. This signal then propagates poleward and downward and is amplified by altered planetary wave activity [8] before being communicated throughout the depth of the troposphere in the Pacific and Atlantic basins [14] . This mechanism can also drive changes in tropical lower stratosphere temperatures, which can additionally affect the troposphere [15] . There is currently uncertainty regarding the ultraviolet variability that accompanies changes in total solar irradiance (TSI) [16] . Recent satellite measurements from the Spectral Irradiance Monitor (SIM) on the Solar Radiation and Climate Experiment satellite [17] show that the variability in ultraviolet over part of the declining phase of solar cycle 23 might be considerably larger than indicated by previous estimates [17] , [18] . Here, our experiments aim to explore the impact of this uncertainty in ultraviolet in the future Maunder Minimum scenario [2] , using both Naval Research Laboratory Spectral Solar Irradiance model output [19] and the SIM data as a basis to estimate lower (EXPT-A) and upper (EXPT-B) bounds for the change in ultraviolet. Regional structure is found in the wintertime response in both experiments, with enhanced relative cooling over northern Eurasia and the eastern United States. For EXPT-B, the change in winter northern European surface temperatures over the late twenty-first century is found to be of similar magnitude to the difference between RCP6.0 and RCP4.5 projections for this region. We conclude that solar forcing may be an important source of uncertainty in regional climate projections. Solar forcing scenarios The future solar forcing scenarios are imposed on an ocean–atmosphere climate model following the representative concentration pathway (RCP) 8.5 for the period 2005 to 2100. Information on the model, experiment ensemble sizes and details of the construction of the solar forcing scenarios can be found in Methods. The scenarios are illustrated in Fig. 1 , which shows the time variation in TSI and ultraviolet irradiance (defined here to be in the range 200–320 nm) for the control (hereafter CTRL-8.5) and experiments with respect to the mean of CTRL-8.5. The mean difference relative to the repeated solar cycle in CTRL-8.5 is a reduction in TSI of 1.74 W m −2 (0.127%) for EXPT-A and 1.76 W m −2 (0.129%) for EXPT-B. For the ultraviolet component, the reduction is 0.25 W m −2 (0.91%) for EXPT-A and 1.76 W m −2 (6.43%) for EXPT-B. 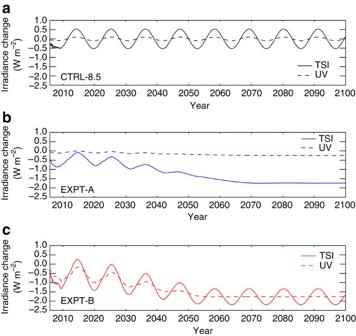Figure 1: Future solar forcing scenarios. Variations in solar forcing for Total Solar Irradiance (W m−2) and ultraviolet irradiance in the 200–320 nm spectral band (W m−2) relative to the mean of the repeated cycle in CTRL-8.5 for (a) CTRL-8.5 (black), (b) EXPT-A (blue) and (c) EXPT-B (red). The value of this mean is 1,366.2 W m−2for TSI and 27.4 W m−2for the ultraviolet band. Figure 1: Future solar forcing scenarios. Variations in solar forcing for Total Solar Irradiance (W m −2 ) and ultraviolet irradiance in the 200–320 nm spectral band (W m −2 ) relative to the mean of the repeated cycle in CTRL-8.5 for ( a ) CTRL-8.5 (black), ( b ) EXPT-A (blue) and ( c ) EXPT-B (red). The value of this mean is 1,366.2 W m −2 for TSI and 27.4 W m −2 for the ultraviolet band. Full size image Global mean temperature response As a result of the decrease in solar irradiance, both experiments show widespread cooling with respect to CTRL-8.5 ( Fig. 2 ). The relative annual global mean near-surface temperature change for the period 2050–2099 is a cooling of 0.13 and 0.12 °C for EXPT-A and EXPT-B, respectively. This offsets or delays the global warming trend by ∼ 2 years and is small compared with the modelled global warming. This is consistent with other recently published results [3] , [4] , [5] , [6] , [7] , which indicate that any change in global mean temperature due to a future prolonged solar minimum would do little to substantially offset or delay the warming due to projected increases in long-lived greenhouse gases. A comparison of forcings and responses can be found in ref. 20 . In some of these studies, potential for regional variation is indicated [4] , [6] , [7] , and we now explore this in more detail in our experiments. 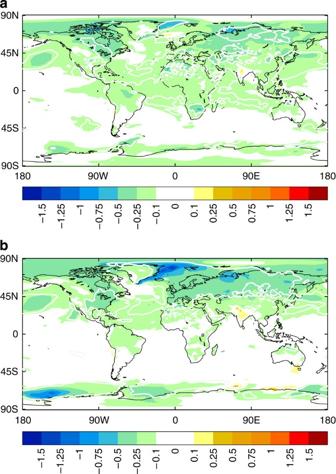Figure 2: Annual mean surface temperature response for future solar experiments. Difference in near-surface temperature (°C) between (a) EXPT-A and (b) EXPT-B and CTRL-8.5 for the period 2050–2099. Solid white contours indicate significance with a 95% confidence interval. Figure 2: Annual mean surface temperature response for future solar experiments. Difference in near-surface temperature (°C) between ( a ) EXPT-A and ( b ) EXPT-B and CTRL-8.5 for the period 2050–2099. Solid white contours indicate significance with a 95% confidence interval. Full size image Northern hemisphere winter response In our experiments, while cooling is evident year round, the largest and most coherent anomalies are in the northern hemisphere in boreal winter and spring. Much of this structure can be explained by a relative change in atmospheric circulation. During December to February, a negative AO/NAO-like mean sea-level pressure pattern is seen in both experiments ( Fig. 3a,e ). Over the North Pacific, the deepened Aleutian low is consistent with the observed pressure response to changes in solar activity [10] , [21] , [22] . In the Atlantic sector, EXPT-B has a stronger and more significant response, showing a weakening in the NAO (defined for the model as the difference in sea-level pressure between gridpoints nearest to the Azores and southwest Iceland) of 1.8 hPa, which is a notable proportion of the interannual standard deviation of 7–8 hPa. Again, the NAO pattern is consistent with the observed response associated with the 11-year cycle over the recent re-analysis period [11] , which has been found to be significant and maximizes at a lag of ∼ 3–4 years for the period 1870–2010 (ref. 10 ). Relative to the historical control period (1971–2000), CTRL-8.5 has a negative shift in the NAO with a significant decrease of 3.2 hPa for the period 2050–2099 (not shown). This is broadly consistent with other modelling studies where the models have well resolved stratospheres [23] , [24] . 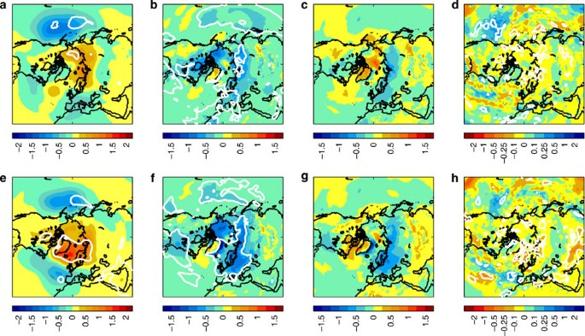Figure 3: Winter climate response for future solar minimum experiments. Differences between experiments and CTRL-8.5 for the period 2050–2099 for (a,e) sea-level pressure (hPa), (b,f) near-surface temperature (°C), (d,h) precipitation (mm day−1). (c,g) They are as inbandfbut with control lagged by 2 years to give similar global mean temperature. Upper panel plots are for EXPT-A and lower panel plots are for EXPT-B. Anomalies are for December to February. Solid white contours indicate significance with a 95% confidence interval. Figure 3: Winter climate response for future solar minimum experiments. Differences between experiments and CTRL-8.5 for the period 2050–2099 for ( a , e ) sea-level pressure (hPa), ( b , f ) near-surface temperature (°C), ( d , h ) precipitation (mm day −1 ). ( c , g ) They are as in b and f but with control lagged by 2 years to give similar global mean temperature. Upper panel plots are for EXPT-A and lower panel plots are for EXPT-B. Anomalies are for December to February. Solid white contours indicate significance with a 95% confidence interval. Full size image There are marked regional differences in the wintertime pattern of cooling in the northern hemisphere with enhanced cooling over northern Eurasia and in the eastern U.S. in both experiments ( Fig. 3b,f ). Average temperature changes for northern hemisphere geographic regions [25] ( Table 1 ) show overall cooling, but with significant and larger or comparable cooling for EXPT-B in the above regions consistent with the stronger negative NAO/AO in this experiment. Cooling to the east of Greenland in EXPT-B, and to a lesser extent in EXPT-A, is associated with a relative increase in the southward transport of sea ice by the East Greenland current (not shown); however, the observed relationship between the NAO and East Greenland sea ice is thought to be epoch dependent [26] , and different models show a range of such relationships [27] , so this element of our model’s response may not be robust. Table 1 Regional winter temperature response. Full size table The quadrupole surface temperature response associated with a decrease in the AO/NAO [28] is evident when the global warming spatial pattern, defined for the purposes of this demonstration as the mean temperature in CTRL-8.5 at a lag of 2 years, has been removed ( Fig. 3c,g ). The general pattern of warming over northeastern North America/Greenland and southern Europe/northern Africa and cooling over southeastern North America and northern Europe can be seen more clearly in EXPT-B ( Fig. 3g ). Analysis of the stratospheric circulation [20] indicates that these changes are associated with a ‘top-down’ stratospheric pathway, as identified in a number of solar studies [8] , [9] , [12] . In EXPT-B, precipitation ( Fig. 3h ) increases in a wide band across the Atlantic and southern parts of Europe, extending eastwards across the Eurasian continent. There are decreases in precipitation over northern Europe. In general, EXPT-A ( Fig. 3d ) shows a similar but noisier response, with less significant signals. These changes are associated with a southward shift of the jet stream and decreased (increased) blocking over southern (northern) Europe in the experiments [20] . Changes in the frequency of extreme events are also affected. CTRL-8.5 shows a large decrease in frost days (20–35 days per winter) over much of southern and central Europe, northern Africa and southeast US for 2050–2099 relative to the historical simulation (1971–2000). There are also large changes over sea areas on the Canadian east coast and to the east of Greenland associated with the retreat of sea ice owing to anthropogenic climate change ( Fig. 4a ). In EXPT-B ( Fig. 4c ), and to a lesser extent in EXPT-A ( Fig. 4b ), we can see the clear signature of the negative AO/NAO with increases of a few frost days per winter in northern Europe and southeast US relative to CTRL-8.5, again consistent with NAO variability on other timescales [29] . 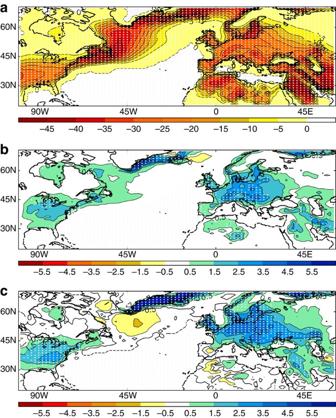Figure 4: Change in average number of frost days. Difference in winter (December to February) frost days (days) between (a) CTRL-8.5 (2050–2099) and the historical period (1971–2000), (b) EXPT-A and CTRL-8.5 (2050–2099) and (c) EXPT-B and CTRL-8.5 (2050–2099). Here, frost days correspond to a daily minimum surface air temperature <0 °C. White stippling indicates significance with a 95% confidence interval. Figure 4: Change in average number of frost days. Difference in winter (December to February) frost days (days) between ( a ) CTRL-8.5 (2050–2099) and the historical period (1971–2000), ( b ) EXPT-A and CTRL-8.5 (2050–2099) and ( c ) EXPT-B and CTRL-8.5 (2050–2099). Here, frost days correspond to a daily minimum surface air temperature <0 °C. White stippling indicates significance with a 95% confidence interval. Full size image European winter response Examining the European response in more detail, average temperature changes for a northern European region are shown in Fig. 5 . Relative to the historical period (1971–2000), RCP4.5 and CTRL-8.5 show substantial warming with a mean difference for 2050–2099 of 4.1 °C and 6.6 °C, respectively. EXPT-A and EXPT-B follow the same trajectory as CTRL-8.5, but with a reduced warming. Relative to CTRL-8.5, we find decreases in regional temperature for 2050–2099 of 0.4 °C (EXPT-A) and nearly 0.8 °C (EXPT-B). This regional cooling is therefore a notable fraction, ∼ 30% for EXPT-B, of the difference between the temperature changes for CTRL-8.5 and RCP4.5. Indeed, compared with temperature changes for a more comprehensive range of scenarios run using a closely related model [30] , the difference between CTRL-8.5 and EXPT-B is similar to the difference between RCP6.0 and RCP4.5 for this region ( Fig. 5 , inset). 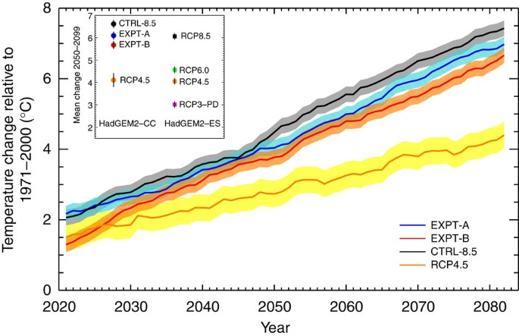Figure 5: Winter European surface temperature response. Mean winter (December to February) northern European (10° W–40° E, 48–75° N) near-surface temperature change (°C, land points only) for 2050–2099 for future scenarios relative to the historical simulation (1971–2000). Shading shows the standard error. The data has been smoothed by applying a 33-year running mean. The inset shows mean winter northern European near-surface temperature differences for 2050–2099 relative to 1971–2000 for the current experiments and for a range of RCP scenarios run with the closely related HadGEM2-ES model30. Whiskers show s.e. Figure 5: Winter European surface temperature response. Mean winter (December to February) northern European (10° W–40° E, 48–75° N) near-surface temperature change (°C, land points only) for 2050–2099 for future scenarios relative to the historical simulation (1971–2000). Shading shows the standard error. The data has been smoothed by applying a 33-year running mean. The inset shows mean winter northern European near-surface temperature differences for 2050–2099 relative to 1971–2000 for the current experiments and for a range of RCP scenarios run with the closely related HadGEM2-ES model [30] . Whiskers show s.e. Full size image Both RCP4.5 and CTRL-8.5 show significant increases in winter precipitation for northern Europe for 2050–2099 relative to the historical period, with a 12% increase for CTRL-8.5 ( Fig. 6a ). As expected with the more negative NAO-like pattern in the solar scenarios, the associated southward shift in the storm track acts to oppose this trend, with both EXPT-A and EXPT-B showing a relative decrease in precipitation compared with CTRL-8.5. In addition, the more southerly storm track enhances precipitation for southern Europe which tends to lessen the drying trend in this region in RCP4.5 and CTRL-8.5 ( Fig. 6b ). The CMIP5 multi-model ensemble projects drying for the Mediterranean region [31] , so in this sensitive region, wintertime alleviation is likely to be important. However, we note that the changes in this region are small and the confidence is relatively low. As with temperature, the changes in precipitation associated with the solar scenarios, are again large fractions of the absolute difference between CTRL-8.5 and RCP4.5; ∼ 65% for northern Europe and 90% for southern Europe in EXPT-B, although the uncertainty for southern Europe is large. 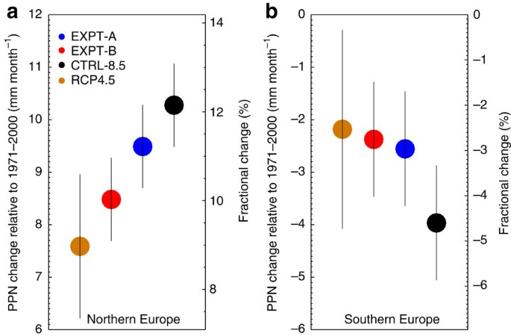Figure 6: Winter European precipitation response. Mean winter (December to February) European precipitation change (mm month−1) for 2050–2099 for future scenarios relative to the historical simulation (1971–2000) for (a) northern Europe (10° W–30° E, 45–65° N) and (b) southern Europe (10° W–30° E, 35–45° N). Whiskers show the s.e. Differences between EXPT-B and CTRL-8.5 are significant with a 90% (75%) confidence interval for northern Europe (southern Europe). Figure 6: Winter European precipitation response. Mean winter (December to February) European precipitation change (mm month −1 ) for 2050–2099 for future scenarios relative to the historical simulation (1971–2000) for ( a ) northern Europe (10° W–30° E, 45–65° N) and ( b ) southern Europe (10° W–30° E, 35–45° N). Whiskers show the s.e. Differences between EXPT-B and CTRL-8.5 are significant with a 90% (75%) confidence interval for northern Europe (southern Europe). Full size image We note that low solar activity does not guarantee cold conditions in any specific European winter as additional variability is introduced by other factors. The 360-year Central England Temperature record for December–February shows that the coldest winters in the UK occurred at low solar activity, but, for example, 1685/6, near the centre of the Maunder minimum, was the 5th warmest winter in the entire record [32] . This highlights the fact that solar variability acts only to bias the intrinsic year-to-year variability, which remains substantial for this region [33] . An example of this from all simulations is that for 12 of the 50 individual years in the period 2050–2099, the warmest ensemble member for northern European winter comes from EXPT-B ( Fig. 7 ). 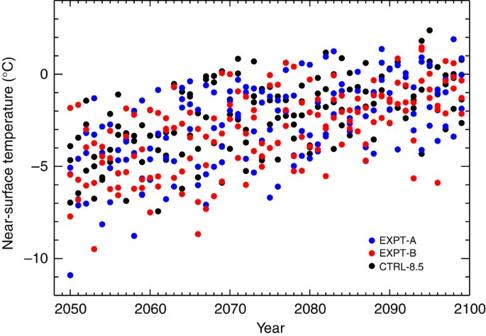Figure 7: Variability in modelled European winter temperatures. Winter (December to January) northern European (10° W–40° E, 48–75° N) near-surface temperatures (°C, land points only) for 2050 to 2099 for individual ensemble members of EXPT-A (blue), EXPT-B (red) and CTRL-8.5 (black). Figure 7: Variability in modelled European winter temperatures. Winter (December to January) northern European (10° W–40° E, 48–75° N) near-surface temperatures (°C, land points only) for 2050 to 2099 for individual ensemble members of EXPT-A (blue), EXPT-B (red) and CTRL-8.5 (black). Full size image Possible feedback mechanisms It has been suggested that solar variability may have affected past variations in North Atlantic temperature and salinity [34] . A positive ocean–atmosphere feedback on the cold northern European temperatures could occur through altered Atlantic heat content [35] and we see a clear signal of a reduced meridional surface temperature gradient over the west North Atlantic for EXPT-B ( Fig. 3f ). Feedbacks could also occur through decreased Atlantic meridional overturning circulation (AMOC) associated either with the persistent negative NAO forcing [36] or with more complex sea ice–ocean–atmosphere mechanisms [37] , [38] , [39] . However, there is uncertainty in the sign of the AMOC response to declining solar activity, with two recent studies suggesting a relative strengthening, associated with weaker radiative forcing and a possible change in stratosphere–troposphere coupling [6] or increased evaporation and densification in the North Atlantic [40] . In our experiments, we find little appreciable change in the AMOC relative to the anthropogenically forced decreasing trend in CTRL-8.5 (not shown). Both experiments show significant changes in tropical precipitation associated with shifts in the Intertropical Convergence Zone, with a southward shift in the Atlantic. These changes are of a pattern and magnitude that has been shown elsewhere [41] to be capable of inducing a compensating strengthening of the AMOC of the magnitude required to balance the effects of negative NAO forcing. However, detailed analysis of the mechanisms of AMOC response is beyond the scope of this paper. Numerous studies have identified links between past climate and solar variability [42] , [43] . During the Maunder Minimum (1645-1715), very few sunspots were seen despite regular observations [44] . If the past relationships between TSI and ultraviolet irradiance and sunspots are the same as are observed for modern solar variability, then a decline in both TSI and ultraviolet for this period can be assumed. The Maunder Minimum coincided with more severe winters in the UK and continental Europe [32] and many reconstructions [45] , [46] suggest atmospheric conditions were broadly comparable with the regional effects on European atmospheric circulation found here. Some modelling studies [13] , [47] also support the idea that similar regional cooling and circulation changes occurred during this period. On longer timescales, cosmogenic isotopes provide a proxy for TSI variations and only indirect meteorological information is available, nevertheless linkages can be made. For example, lake sediments have been analysed to demonstrate that a grand minimum of solar activity, the Homeric Minimum ( ∼ 2,750–2,550 years before present), affected climate conditions through western Europe through altered regional circulation consistent with the negative phase of the NAO [48] . While these paleoclimatic studies appear largely consistent with our model result that weak solar ultraviolet irradiance can have a significant impact on European winter circulation through ‘top-down’ dynamical forcing, detailed modelling and attribution for these events is beyond the scope of this paper. We note that, to date, a variety of strengths of model response for past events have been obtained [13] , [47] , [49] , which could, in part, be related to uncertainties in solar forcing and to the efficiency of the ‘top-down’ mechanism in different models [14] . We note that there are some uncertainties in our model response to solar forcing. The peak-to-trough variability in global mean temperature for the 11-year solar cycle is ∼ 0.06 °C but observational estimates suggest this may be too small. For example, a signal of ∼ 0.1 °C was obtained using a multivariate analysis with up-to-date estimates of natural (including volcanic aerosols) and anthropogenic forcing [50] . In general, climate models appear to underestimate this variability [5] . The modelled Atlantic atmospheric circulation response may also be larger if, as has recently been suggested, the ocean feedback is underestimated in the model [35] . The changes in TSI that are applied in our experiments are representative of current scientific understanding [31] and are smaller than those reported in earlier IPCC reports. The ultraviolet changes are designed to bracket the current uncertainty in spectral irradiance at these wavelengths, but we note that EXPT-B is likely to be at the high end of any estimate of ultraviolet change and the appreciable changes in climate that we find should therefore be viewed as a high estimate in this respect. This research highlights the need for accurate and long-term measurements of spectral solar irradiance to reduce current uncertainties. In the solar scenario presented here, there is a gradual descent to Maunder Minimum-like conditions, which are then maintained for a period of 50 years until the end of the experiment. A modelling study which includes representation of the end of a solar minimum [7] indicates that global mean temperatures approach the reference model climatology within a few years of a return to the reference solar forcing. Although timescales may depend on the exact details of the forcing scenario and model, we would expect a reversal of the climate impacts described in our experiment following the end of the event. Estimates of the duration of grand solar minima, based on model reconstruction from 14 C data [51] and from 10 Be data [52] , vary from a few decades to more than 100 years [53] . The latest data [1] (updated October 2013) on sunspot number, near-Earth interplanetary conditions, cosmic ray fluxes and geomagnetic activity are all consistent with the most rapid fall scenario used here [2] . All these data are in the upper 5 percentile of the distributions (lower 5 percentile in the case of cosmic rays which anti-correlate with solar activity) of predictions extended to these parameters [53] . Note also that these statistical predictions [51] are very similar to the predictions made using spectral techniques [54] . Thus all the current indicators are consistent with the most extreme decline discussed by Lockwood [2] . However, it should be remembered these predictions are statistical and not physical in nature, being based on past behaviour. The northern hemisphere winter regional temperature and precipitation changes associated with the reduced solar forcing can amount to a substantial fraction of the difference between plausible RCP scenarios. Our results therefore suggest that uncertainties in natural forcing, in this case both the uncertainty in future solar output and uncertainty in spectral solar irradiance, should be taken into account alongside uncertainties in emissions in future climate forcing scenarios. The control model We use the Met Office Hadley Centre general circulation model, HadGEM2-CC (carbon cycle) [55] , with historical and future forcings specified according to the Fifth Coupled Model Intercomparison Project (CMIP5) as used in HadGEM2-ES (Earth System) [30] . This version of HadGEM2 is a ‘high top’ model with 60 vertical levels and an upper boundary at 84 km, so is capable of resolving relevant stratospheric processes [56] , [57] , [58] . The horizontal resolution is 1.875° longitude by 1.25° latitude. The ocean resolution is 1° × 1°, increasing in the tropics to 0.3°, with 40 vertical levels. The TSI is partitioned across six shortwave spectral bands (0.2–10 μm) with spectral changes associated with changing TSI accounted for. For the historical period, the TSI and spectrally resolved irradiance (SSI) used is that recommended by CMIP5 (Lean, Calculations of solar irradiance, http://sparcsolaris.gfz-potsdam.de/cmip5.php , accessed 2 June 2009 from the earlier fuberlin site), with a repeating 11-year cycle, based on the period 1998–2008, imposed for future scenarios. Time-varying ozone distributions include a component related to solar variability [30] . Grand solar minimum scenario The solar forcing is based on the most rapidly declining Lockwood [2] solar activity scenario and uncertainty in future levels of ultraviolet is explored with two experiments designed to bracket uncertainty in ultraviolet spectral irradiance. Experiments are initialized from 1 December 2005 with the same initial conditions as the parallel CTRL-8.5 ensemble. The derivation of the forcing is as follows: EXPT-A The future TSI for EXPT-A is constructed by relating changes in the historical TSI to the past solar modulation parameter, then applying this relationship to the future scenario for the parameter [1] , [2] . The SSIs are calculated by extrapolation of second-order polynomial fits of SSI versus TSI from the CMIP5 historical forcing data set. This experiment describes a relatively modest change in ultraviolet. The solar component in the prescribed ozone field also scales with the change in TSI. EXPT-B For EXPT-B, 200–320 nm data from the SIM instrument (2004–2009) are fitted to a typical solar cycle shape, giving an estimate for a peak-to-trough change in ultraviolet of 1.17 W m −2 . The SIM data used in this study is based on more reliable SORCE SIM Version 17 processing, but these results are consistent with the published version, Version 22, available at: http://lasp.colorado.edu/home/sorce/data/ . Next, a scaling factor is derived between the Open Solar Flux (OSF) measure of solar activity [1] , [2] and ultraviolet. It is important to note that the use of the OSF proxy introduces a secular change in the past (and predicted future) ultraviolet irradiance that would not be obtained if other solar activity indices (such as the F10.7 radio flux) were used: however, ultraviolet-driven changes in the stratosphere are more highly correlated with OSF than indices such as F10.7 that do not show the same secular trends [59] . The scaling used here is based on calculating the average of peak-to-trough values in de-trended OSF data for the period 1982–2008 and taking this average to be equal to the SIM data estimate giving a relationship of 2.19 OSF units equalling 1 W m −2 of ultraviolet irradiance. The future projection in ultraviolet forcing is calculated by scaling the OSF for the grand solar minimum scenario, deriving a change in ultraviolet irradiance that would be consistent with the SIM data scaling linearly with the assumed future trend in OSF. The baseline period for normalizing the OSF with respect to the HadGEM2-CC historical forcing is 1964–2008. In EXPT-B, only the ultraviolet (200–320 nm) component of the shortwave irradiance is adjusted. Radiation bands 2 to 6 are unaltered, and so retain variability on the 11-year timescale out to 2100. This means that the reduction in TSI is by definition equal to the reduction in ultraviolet. In this experiment, the prescribed ozone is the same as that in CTRL-8.5. This enables direct comparison of the impact of UV changes with CTRL-8.5 and we believe it is justified as the large change in ultraviolet is likely to dominate the change in stratospheric heating in this case. We might expect inclusion of interactive ozone to enhance the response, but think this is likely to be of secondary importance for EXPT-B. However, we note that GCM studies have shown sensitivity to the magnitude and distribution of specified ozone changes [22] , [60] . Ensemble sizes and experiments used for comparison HadGEM2-CC: CTRL-8.5, EXPT-B and EXPT-A have three ensemble members, while RCP4.5 has just a single member. The historical runs have three ensemble members. HadGEM2-ES: All RCPs and historical runs have four ensemble members. All the results are for ensemble means, unless otherwise stated. Statistics Model statistical significance is tested using the Mann–Whitney test (a nonparametric test) with the null hypothesis that the difference in means are not significantly different from zero. One-tailed tests are used, given the prior evidence for a negative AO/NAO response [8] , [10] . Code availability Due to intellectual property right restrictions, we cannot provide either the source code or the documentation papers for HadGEM2. The Met Office Unified Model (MetUM) is available for use under licence. A number of research organizations and national meteorological services use the MetUM in collaboration with the Met Office to undertake basic atmospheric process research, produce forecasts, develop the MetUM code and build and evaluate Earth system models. For further information on how to apply for a licence, see http://www.metoffice.gov.uk/research/collaboration/um-collaboration . How to cite this article: Ineson, S. et al. Regional climate impacts of a possible future grand solar minimum. Nat. Commun. 6:7535 doi: 10.1038/ncomms8535 (2015).